Ecophysiology and interactions of a taurine-respiring bacterium in the mouse gut 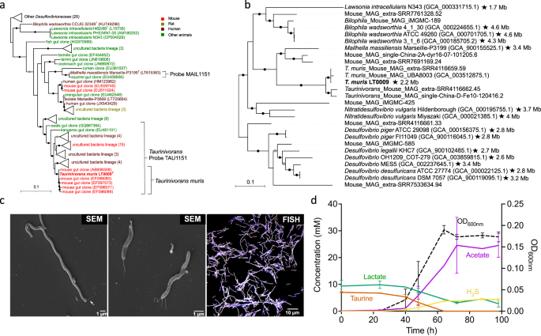Fig. 1: Phylogeny and morphology of the mouse gut-derived taurine-respiring strain LT0009 that represents the new genus/speciesTaurinivorans murisin the familyDesulfovibrionaceae. a16 S rRNA gene tree and FISH probe coverage. Maximum likelihood branch supports (1000 resamplings) equal to or greater than 95% and 80% are indicated by black and gray circles, respectively. The scale bar indicates 0.1 estimated substitutions per residue. Accession numbers are shown in parentheses. Strain LT0009 is shown in bold and type strains are marked with a superscript ‘T’. Sequence sources are indicated with different colors (Supplementary Data2). Sequences were assigned toTaurinivoransandTaurinivorans murisbased on the genus-level similarity cutoff of 94.5% and species-level similarity cutoff of 98.7%106, respectively. The perfect-match coverage of probes TAU1151 forTaurinivoransand MAIL1151 forMailhellais indicated.bPhylogenomic tree. Ultrafast bootstrap support values equal to or greater than 95% and 80% for the maximum likelihood tree are indicated with black and gray circles, respectively. Accession numbers are shown in parentheses. Strain LT0009 is shown in bold. Strains with complete genomes (genome size is indicated) are marked with a star. Genomes were assigned toTaurinivoransbased on the genus-level AAI cutoff value of 63.4%107. The scale bar indicates 0.1 estimated substitutions per residue.cRepresentative morphology of LT0009 cells in pure culture (n= 3 independent cultures). SEM: Scanning electron microscopy images of cells of varying lengths. White arrows indicate the flagella. FISH: Cells hybridized with Cy3-labeled probe TAU1151 and Fluos-labeled probe EUB338mix and counterstained by DAPI.dGrowth of strain LT0009 in modifiedDesulfovibriomedium confirmed complete utilization of taurine as electron acceptor concomitant with nearly stoichiometric production of sulfide. Electron donors L-lactate and pyruvate were provided in excess, and their utilization also contributed to acetate formation. Pyruvate in the medium and ammonia released from the deamination of taurine were not analyzed in this experiment. Lines represent averages of measures in triplicate cultures. Error bars represent one standard deviation (n= 3 biologically independent cultures). Source data are provided as a Source Data file. Taurine-respiring gut bacteria produce H 2 S with ambivalent impact on host health. We report the isolation and ecophysiological characterization of a taurine-respiring mouse gut bacterium. Taurinivorans muris strain LT0009 represents a new widespread species that differs from the human gut sulfidogen Bilophila wadsworthia in its sulfur metabolism pathways and host distribution. T. muris specializes in taurine respiration in vivo, seemingly unaffected by mouse diet and genotype, but is dependent on other bacteria for release of taurine from bile acids. Colonization of T. muris in gnotobiotic mice increased deconjugation of taurine-conjugated bile acids and transcriptional activity of a sulfur metabolism gene-encoding prophage in other commensals, and slightly decreased the abundance of Salmonella enterica , which showed reduced expression of galactonate catabolism genes. Re-analysis of metagenome data from a previous study further suggested that T. muris can contribute to protection against pathogens by the commensal mouse gut microbiota. Together, we show the realized physiological niche of a key murine gut sulfidogen and its interactions with selected gut microbiota members. Hydrogen sulfide (H 2 S) is an intestinal metabolite with pleiotropic effects, particularly on the gut mucosa [1] , [2] . H 2 S can have a detrimental impact on the intestinal epithelium by chemically disrupting the mucus barrier [3] , causing DNA damage [4] , and impairing energy generation in colonocytes through inhibiting cytochrome c oxidase and beta-oxidation of short-chain fatty acids [5] , [6] . In contrast, low micromolar concentrations of H 2 S are anti-inflammatory and contribute to mucosal homeostasis and repair [7] , [8] . Furthermore, H 2 S acts as a gaseous transmitter, a mitochondrial energy source, and an antioxidant in cellular redox processes. Thus, its impact on mammalian physiology and health reaches beyond the gastrointestinal tract [9] . For example, colonic luminal H 2 S can promote somatic pain in mice [10] and contribute to regulating blood pressure [11] , [12] . The multiple (patho)physiological functions of H 2 S in various organs and tissues depend on its concentration and the host’s health status, but possibly also on the source of H 2 S. Mammalian cells can produce H 2 S from cysteine via several known pathways [13] . In contrast to these endogenous sources, H 2 S-releasing drugs and H 2 S-producing intestinal microorganisms are considered exogenous sources. Sulfidogenic bacteria, which either metabolize organic sulfur compounds (e.g., cysteine) or anaerobically respire organic (e.g., taurine) or inorganic (e.g., sulfate, sulfite, tetrathionate) sulfur compounds in the gut, have a higher H 2 S-producing capacity and are thus potentially harmful to their hosts [1] , [2] , [14] . Indeed, the abundance and activity of sulfidogenic gut bacteria were associated with intestinal diseases such as inflammatory bowel disease and colon cancer in various studies [15] , [16] , [17] and many gut pathogens, such as Salmonella enterica and Clostridioides difficile , are also sulfidogenic [18] , [19] . Excess bacterial H 2 S production combined with a reduced capacity of the inflamed mucosa to metabolize H 2 S is one of many mechanisms by which the gut microbiome can contribute to disease [20] . Yet, the manifold endogenous and microbial factors and processes that regulate intestinal H 2 S homeostasis are insufficiently understood. A major and constantly available substrate of sulfidogenic bacteria in the gut is the organosulfonate taurine (2-aminoethanesulfonate). Taurine derives directly from the host’s diet, in highest amounts from meat and seafood and to a lower extent from algae and plants [21] , but is also liberated by microbial bile salt hydrolases (BSHs) from endogenously produced taurine-conjugated bile acids [22] . Bilophila wadsworthia is the most prominent taurine-utilizing bacterium in the human gut. Diets that contain high quantities of meat, dairy products, or fats can be associated with the outgrowth of B. wadsworthia in the gut [23] , [24] . Consumption of high-fat food triggers taurine-conjugated bile acid production and increases the taurine:glycine ratio in the bile acid pool [24] . In mouse models, higher abundances of B. wadsworthia can promote colitis and systemic inflammation [24] , [25] and aggravate metabolic dysfunctions [26] . B. wadsworthia metabolizes taurine via the two intermediates sulfoacetaldehyde and isethionate (2-hydroxyethanesulfonate) to sulfite [27] , and the sulfite is utilized as electron acceptor for energy conservation and reduced to H 2 S via the DsrAB-DsrC dissimilatory sulfite reductase system [28] . The highly oxygen-sensitive isethionate sulfite-lyase system IslAB catalyzes the abstraction of sulfite (desulfonation) of isethionate [27] , [29] . Alternative taurine degradation pathways in other bacteria involve direct desulfonation of sulfoacetaldehyde by the oxygen-insensitive, thiamine-diphosphate-dependent sulfoacetaldehyde acetyltransferase Xsc [30] , [31] , [32] . Xsc is employed (i) in taurine utilization pathways of a wide range of aerobic bacteria that use taurine as carbon and energy source [31] , [33] , and (ii) for anaerobic taurine fermentation by Desulfonispora thiosulfatigenes [32] . Here, we isolated a taurine-respiring and H 2 S-producing bacterium from the murine intestinal tract and elucidated its fundamental and in vivo realized nutrient niche. We show that strain LT0009 represents a new Desulfovibrionaceae genus, for which we propose the name Taurinivorans muris gen. nov., sp. nov., and differs from its human counterpart B. wadsworthia by using the Xsc pathway for taurine degradation and its distribution across different animal hosts. We further provide initial insights into the protective role of T. muris against pathogen colonization. A taurine-respiring bacterium isolated from the murine gut represents a new genus of the family Desulfovibrionaceae Strain LT0009 was enriched from mouse cecum and colon using an anoxic, non-reducing, modified Desulfovibrio medium with L-lactate and pyruvate as electron donors (and carbon source) and taurine as the sulfite donor for sulfite respiration. Its isolation was achieved by several transfers in liquid medium, purification by streaking on ferric-iron supplemented agar plates, indicating sulfide production by black FeS formation and picking of black colonies, and by additional purification using dilution-to-extinction in liquid medium. We sequenced and reconstructed the complete LT0009 genome, which has a size of 2.2 Mbp, a G + C content of 43.6%, and is free of contamination as assessed by CheckM [34] . The genome comprises 2,059 protein-coding genes (Supplementary Data 1 ), 56 tRNA genes, 4 rRNA operons (with 5 S, 16 S, and 23 S rRNA genes), 4 pseudogenes, and 6 miscellaneous RNA genes. LT0009 formed a monophyletic, genus-level (>94.5% similarity) lineage with other 16 S rRNA gene sequences from the gut of mice and other hosts. It has <92% 16 S rRNA gene sequence identity to the closest related strains Marseille-P3669 and Mailhella massiliensis Marseille-P3199 T that were isolated from human feces (Fig. 1a ). Phylogenomic treeing and an AAI of <60% to other described species strongly suggested that LT0009 represents the type strain of a novel genus in the family Desulfovibrionaceae of the phylum Desulfobacterota [35] for which we propose the name Taurinivorans muris (Fig. 1b , Supplementary Fig. 1 , Supplementary Information). The previously described mouse gut MAGs UBA8003 and extra-SRR4116659.59 have >98% ANI and AAI to LT0009 and thus also belong to the species T. muris [36] , [37] , [38] . Furthermore, the mouse gut MAGs extra-SRR4116662.45 and single-China-D-Fe10-120416.2 showed 79% AAI/ANI to strain LT0009 and 84% AAI and 82% ANI to each other, which indicates that each of these two MAGs would likely represent a separate species in the genus Taurinivorans . Notably, the genome of T. muris LT0009 with only 2.2 Mbp in size is considerably smaller and thus potentially more streamlined than those of other free-living bacteria of the Desulfovibrio-Bilophila-Lawsonia-Mailhella -lineage (Fig. 1b ). Only the obligate intracellular intestinal pathogen Lawsonia intracellularis has a smaller genome at 1.5-1.7 Mbp [39] , [40] . Fig. 1: Phylogeny and morphology of the mouse gut-derived taurine-respiring strain LT0009 that represents the new genus/species Taurinivorans muris in the family Desulfovibrionaceae . a 16 S rRNA gene tree and FISH probe coverage. Maximum likelihood branch supports (1000 resamplings) equal to or greater than 95% and 80% are indicated by black and gray circles, respectively. The scale bar indicates 0.1 estimated substitutions per residue. 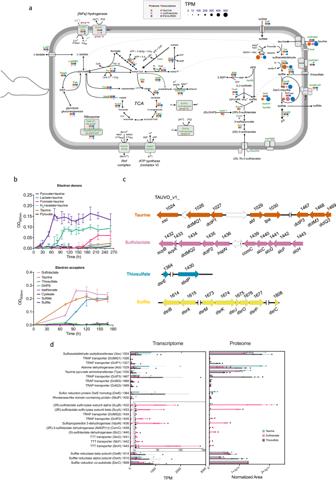Fig. 2: Sulfur-based energy metabolism ofTaurinivorans murisLT0009. aCell cartoon of the central sulfur and energy metabolism of LT0009 as determined by genome, transcriptome, and proteome analyses. Genes/proteins detected in the transcriptome and proteome of LT0009 grown with taurine, sulfolactate, or thiosulfate as electron acceptor are shown by colored circles and squares, respectively. Circle size indicates gene transcription level normalized as TPM. Proteins of all transcribed genes were also detected in the proteome, with the exception of AprAB, TauA (TAU_v1_0027, TAU_v1_1344), TauB, TauC, TauE, DctMQ2, SlcG, DsrEFH, AscA, two [FeFe] hydrogenases (TAU_v1_1126, TAU_v1_1901), cytochromecand Sdh. Protein complexes (e.g., Rnf, SlcFGH, DctPMQ2, Atp) are not shown with transcriptome and proteome data because at least one gene/protein of the complex units was not detected. The gene annotations are listed in Supplementary Data 7.bAnaerobic growth tests of strain LT0009 with various substrates (n= 3 biologically independent cultures). Electron donors: All substrates were added at 10 mmol/l concentration, except acetate (20 mmol/l), which was added as carbon source together with H2. Electron acceptors: The different sulfur compounds were added at 10 mmol/l concentration together with pyruvate, lactate, and 1,4-naphthoquinone. OD600: optical density at 600 nm.cOrganization of sulfur metabolism genes in the LT0009 genome. Numbers show the RefSeq locus tag with the prefix TAUVO_v1.dComparative transcriptome and proteome analysis of LT0009 grown with lactate and taurine, sulfolactate, or thiosulfate as electron acceptor. Numbers following protein names refer to RefSeq locus tag numbers (prefix TAUVO_v1). Protein expression was normalized to DsrC for each growth condition. Bars represent averages and error bars represent one standard deviation (n= 3 biologically independent cultures). Asterisk indicates significant (p< 0.05, exactpvalues are provided in Supplementary Data 1) differences in gene transcription/protein expression compared to growth with taurine (5% false discovery rate, DESeq2 Wald test). TCA, tricarboxylic acid cycle; WL, Wood-Ljungdahl pathway; PEP, phosphoenolpyruvate; DHPS, 2,3-dihydroxypropane-1-sulfonate; TPM, transcripts per million. Source data are provided as a Source Data file. Accession numbers are shown in parentheses. Strain LT0009 is shown in bold and type strains are marked with a superscript ‘T’. Sequence sources are indicated with different colors (Supplementary Data 2 ). Sequences were assigned to Taurinivorans and Taurinivorans muris based on the genus-level similarity cutoff of 94.5% and species-level similarity cutoff of 98.7% [106] , respectively. The perfect-match coverage of probes TAU1151 for Taurinivorans and MAIL1151 for Mailhella is indicated. b Phylogenomic tree. Ultrafast bootstrap support values equal to or greater than 95% and 80% for the maximum likelihood tree are indicated with black and gray circles, respectively. Accession numbers are shown in parentheses. Strain LT0009 is shown in bold. Strains with complete genomes (genome size is indicated) are marked with a star. Genomes were assigned to Taurinivorans based on the genus-level AAI cutoff value of 63.4% [107] . The scale bar indicates 0.1 estimated substitutions per residue. c Representative morphology of LT0009 cells in pure culture ( n = 3 independent cultures). SEM: Scanning electron microscopy images of cells of varying lengths. White arrows indicate the flagella. FISH: Cells hybridized with Cy3-labeled probe TAU1151 and Fluos-labeled probe EUB338mix and counterstained by DAPI. d Growth of strain LT0009 in modified Desulfovibrio medium confirmed complete utilization of taurine as electron acceptor concomitant with nearly stoichiometric production of sulfide. Electron donors L-lactate and pyruvate were provided in excess, and their utilization also contributed to acetate formation. Pyruvate in the medium and ammonia released from the deamination of taurine were not analyzed in this experiment. Lines represent averages of measures in triplicate cultures. Error bars represent one standard deviation ( n = 3 biologically independent cultures). Source data are provided as a Source Data file. Full size image The Gram staining of T. muris LT0009 was negative. FISH imaging of the LT0009 pure culture with a genus-specific 16 S rRNA-targeted probe TAU1151 showed cells with a conspicuous spiral-shaped morphology and considerably varying lengths (1.7–28 µm) (Fig. 1c , Supplementary Data 2 , Supplementary Fig. 2 ). SEM imaging further indicated that LT0009 cells have multiple polar flagella, suggesting that they are motile (Fig. 1c ). Complete utilization of taurine as electron acceptor in modified Desulfovibrio liquid medium with electron donors lactate and pyruvate in excess resulted in production of nearly quantitative amounts of H 2 S and excess acetate (Fig. 1d ). Strain LT0009 in pure culture did not grow in the absence of 1,4-naphthoquinone and yeast extract, indicating an absolute requirement of menaquinone (vitamin K2) and other essential growth factors, respectively. Both growth rate and final growth yields were increased when taurine was provided at 20 and 40 mmol/l concentration in comparison to 10 mmol/l, while growth was inhibited at concentrations ≥60 mmol/l taurine (Supplementary Fig. 3a ). Strain LT0009 grew with a lower growth rate and final growth yield when pyruvate was omitted as additional electron donor (Supplementary Fig. 3b ). Strain LT0009 grew equally well at a pH range of 6–8.5 (Supplementary Fig. 3c ) and temperatures between 27–32 °C, but with reduced final growth yield at 37 and 42 °C (Supplementary Fig. 3d ). No colony formation was observed on agar plates under aerobic conditions, suggesting a strict anaerobic lifestyle of T. muris LT0009. Sulfur and energy metabolism of T. muris LT0009 Based on a genome-inferred metabolism prediction of strain LT0009 (Fig. 2a , Supplementary Data 3 ), we tested its growth with substrates that could serve as energy and sulfur sources in the gut. Fermentative growth with only pyruvate or only taurine, i.e., as both electron donor and acceptor, was not observed. In addition to pyruvate and lactate, LT0009 also used formate as electron donor for growth under taurine-respiring conditions, albeit with an extended lag phase and a lower growth yield. For the alternative electron acceptors tested, LT0009 used 3-sulfolactate and thiosulfate in combination with lactate and pyruvate, but did not grow with 2,3-dihydroxypropane-1-sulfonate (DHPS), isethionate, cysteate, and not with inorganic sulfate or sulfite (Fig. 2b ). Fig. 2: Sulfur-based energy metabolism of Taurinivorans muris LT0009. a Cell cartoon of the central sulfur and energy metabolism of LT0009 as determined by genome, transcriptome, and proteome analyses. Genes/proteins detected in the transcriptome and proteome of LT0009 grown with taurine, sulfolactate, or thiosulfate as electron acceptor are shown by colored circles and squares, respectively. Circle size indicates gene transcription level normalized as TPM. Proteins of all transcribed genes were also detected in the proteome, with the exception of AprAB, TauA (TAU_v1_0027, TAU_v1_1344), TauB, TauC, TauE, DctMQ2, SlcG, DsrEFH, AscA, two [FeFe] hydrogenases (TAU_v1_1126, TAU_v1_1901), cytochrome c and Sdh. Protein complexes (e.g., Rnf, SlcFGH, DctPMQ2, Atp) are not shown with transcriptome and proteome data because at least one gene/protein of the complex units was not detected. The gene annotations are listed in Supplementary Data 7. b Anaerobic growth tests of strain LT0009 with various substrates ( n = 3 biologically independent cultures). Electron donors: All substrates were added at 10 mmol/l concentration, except acetate (20 mmol/l), which was added as carbon source together with H 2 . Electron acceptors: The different sulfur compounds were added at 10 mmol/l concentration together with pyruvate, lactate, and 1,4-naphthoquinone. OD 600 : optical density at 600 nm. c Organization of sulfur metabolism genes in the LT0009 genome. Numbers show the RefSeq locus tag with the prefix TAUVO_v1. d Comparative transcriptome and proteome analysis of LT0009 grown with lactate and taurine, sulfolactate, or thiosulfate as electron acceptor. Numbers following protein names refer to RefSeq locus tag numbers (prefix TAUVO_v1). Protein expression was normalized to DsrC for each growth condition. Bars represent averages and error bars represent one standard deviation ( n = 3 biologically independent cultures). Asterisk indicates significant ( p < 0.05, exact p values are provided in Supplementary Data 1) differences in gene transcription/protein expression compared to growth with taurine (5% false discovery rate, DESeq2 Wald test). TCA, tricarboxylic acid cycle; WL, Wood-Ljungdahl pathway; PEP, phosphoenolpyruvate; DHPS, 2,3-dihydroxypropane-1-sulfonate; TPM, transcripts per million. Source data are provided as a Source Data file. Full size image The metabolic pathways used for growth by respiration with taurine, sulfolactate, or thiosulfate and with lactate/pyruvate as electron donors were further analyzed by both differential transcriptomics and differential proteomics, as transcription and translation can be uncoupled in bacteria [41] , [42] . These analyses and comparative sequence analyses of the key genes/proteins (Supplementary Fig. 4 ) strongly suggested that taurine is degraded via the Tpa-Ald-Xsc pathway and the produced sulfite respired via the DsrAB-DsrC pathway (Fig. 2c, d ). Notably, Tpa, Ald, and Xsc were among the top thirteen most abundant proteins that were detected in strain LT0009 grown with all three electron acceptors (Supplementary Fig. 5 ). Yet, relative protein abundances of Tpa and Ald but not Xsc were significantly increased in cells grown with taurine compared to cells grown with thiosulfate (Fig. 2d ). Pyruvate-dependent taurine transaminase Tpa catalyzes initial conversion of taurine to alanine and sulfoacetaldehyde [32] . Oxidative deamination of alanine to pyruvate is catalyzed by alanine dehydrogenase Ald (Fig. 2a, c, d ). Lack of the sulfoacetaldehyde reductase gene sarD and islAB and inability to grow with isethionate showed that LT0009 does not have the taurine degradation pathway of B. wadsworthia [27] . Instead, sulfoacetaldehyde is directly desulfonated to acetyl-phosphate and sulfite by thiamine-diphosphate-dependent sulfoacetaldehyde acetyltransferase Xsc [30] , [31] , [32] . The acetyl-phosphate is then converted to acetate and ATP by acetate kinase AckA. Strain LT0009 seems to lack candidate genes for the TauABC taurine transporter [43] . While homologs of tauABC are encoded in the genome, the individual genes do not form a gene cluster like in Escherichia coli [44] and were not expressed during growth on taurine (Supplementary Data 1 ). Instead, the LT0009 genome encodes three copies of gene sets for tripartite ATP-independent periplasmic (TRAP) transporter [45] that are co-encoded in the taurine degradation gene cluster and were expressed during growth with taurine, thus are most likely involved in taurine import, including DctPQM1 (with fused DctQM1) (TAUVO_v1_1026 and 1027) and DctPQM3 (TAUVO_v1_1467-1469) (Fig. 2c, d ). (2 S)-3-sulfolactate is degraded by LT0009 via the SlcC-ComC-SuyAB pathway as shown by differential expression of these enzymes in cells grown with racemic sulfolactate (Fig. 2c, d , Supplementary Data 1 ). The dehydrogenases (S)-sulfolactate dehydrogenase SlcC and (R)-sulfolactate oxidoreductase ComC isomerize (2 S)-3-sulfolactate to (2 R)-3-sulfolactate via 3-sulfopyruvate. (2 R)-3-sulfolactate is desulfonated to pyruvate and sulfite by sulfo-lyase SuyAB, which was significantly increased in sulfolactate-grown cells compared to taurine or thiosulfate-grown cells (Fig. 2d ). The neighboring gene clusters slcHFG-slcC-comC and hpsN-dctPQM2-suyAB were both significantly upregulated in the transcriptome of sulfolactate-grown cells (Fig. 2d ). The DctPQM2 (with fused DctQM2) (TAUVO_v1_1434 and 1435) TRAP transporter and the SlcGFH tripartite tricarboxylate transporters (TTT) [45] , [46] are putative sulfolactate importers. The gene cluster further includes a homolog to hpsN , encoding sulfopropanediol-3-dehydrogenase [47] . This enzyme converts (R)-DHPS to (R)-sulfolactate during aerobic catabolism of DHPS by diverse bacteria in soils [54] and the ocean [48] . However, LT0009 did not grow with racemic DHPS when tested (Fig. 2b ). The hpsN gene was transcribed in LT0009 with taurine, sulfolactate, and thiosulfate treatments, but the HpsN protein was not detected (Supplementary Data 1 ). LT0009 did not grow with cysteate as an electron acceptor under the conditions we used, although it encodes a homolog of L-cysteate sulfo-lyase CuyA that desulfonates L-cysteate to pyruvate, ammonium, and sulfite [49] , [50] (Fig. 2b ). Yet, CuyA can also act as D-cysteine desulfhydrase [49] . The cuyA gene was transcribed in the presence of taurine, sulfolactate, and thiosulfate. Furthermore, CuyA was significantly higher expressed in LT0009 with taurine ( P < 0.001) compared with sulfolactate and thiosulfate (Supplementary Data 1 ), yet its physiological role in LT0009 remains unclear. Strain LT0009 respired thiosulfate, such as B. wadsworthia strain RZATAU [51] , but lacks genes for PhsABC thiosulfate reductase [52] and thiosulfate reductase from Desulfovibrio (EC 1.8.2.5) [53] , which both (i) disproportionate thiosulfate to sulfide and sulfite and (ii) are present in the human B. wadsworthia strains ATCC 49260, 4_1_30, and 3_1_6. LT0009 has a gene for a homolog of rhodanese-like, sulfur-trafficking protein SbdP (TAUVO_v1_1430) (Supplementary Fig. 4g ) [54] . Rhodaneses (EC 2.8.1.1.) can function as thiosulfate sulfur transferase and produce sulfite [55] . Homologs of SbdP are broadly distributed in members of the Desulfovibrio-Bilophila-Mailhella-Taurinivorans clade and other Desulfovibrionaceae (Supplementary Fig. 4g ). The SbdP-homolog in LT0009 (TAUVO_v1_1430) could (i) provide sulfite for reduction and energy conservation by the Dsr sulfite reductase system and (ii) transfer the second sulfur atom from thiosulfate to an unknown acceptor protein/enzyme. A candidate sulfur-accepting protein is encoded by a dsrE -like gene in LT0009 (TAUVO_v1_1364) (Supplementary Fig. 4e ). High expression of rhodanese-like sulfur transferases, a DsrE-like protein, and DsrAB sulfite reductase was reported for thiosulfate-respiring Desulfurella amilsii [56] . However, the functions of the SbdP-sulfur transferase and the DsrE-like protein in the thiosulfate metabolism of LT0009 remain unconfirmed. First, these proteins are not homologous to the highly expressed D. amilsii proteins. Second, comparative transcriptome and proteome analyses were inconclusive, as only the transcription of the dsrE -like gene was upregulated in LT0009 grown with thiosulfate (Fig. 2d , Supplementary Data 1 ). Additional genes homologous to known sulfur metabolism genes whose functions in LT0009 remain enigmatic include sudAB , which encode sulfide dehydrogenase for reduction of sulfur or polysulfide to H 2 S [57] , and dsrEFH , which are involved in sulfur atom transfer in sulfur oxidizers (Supplementary Fig. 4f ) [58] . LT0009 encodes an incomplete pathway for dissimilatory sulfate reduction. While homologs of genes for the sulfate transporter SulP [59] and adenylyl-sulfate reductase AprAB were present, the absence of genes for sulfate adenylyltransferase Sat and the electron-transferring QmoAB complex (Supplementary Data 3 ) was consistent with the inability of LT0009 to respire sulfate. Although externally supplied sulfite did not support growth, the DsrAB-DsrC dissimilatory sulfite reductase system was highly expressed in cells grown with taurine, sulfolactate or thiosulfate (Fig. 2a, d , Supplementary Data 1 ). This suggests that intracellularly produced sulfite is respired to sulfide via the DsrAB-DsrC system, which includes the transfer of electrons from the oxidation of electron donors via the membrane quinone pool and the DsrMKJOP complex (Fig. 2a ) [60] . Genome reconstruction of LT0009 suggested the potential to utilize lactate, pyruvate, and H 2 as electron donors (Supplementary Information). We experimentally confirmed that lactate, pyruvate, and formate are used as electron donors for taurine respiration (Fig. 2b ). 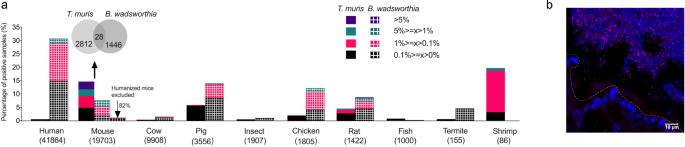Fig. 3:Taurinivorans murisandBilophila wadsworthiahave distinct host distribution patterns. aOccurrence and prevalence ofTaurinivorans muris- andBilophila wadsworthia-related sequences in 16 S rRNA gene amplicon datasets of human and animal guts.T. muris- andB. wadsworthia-like sequences at 97% similarity cutoff are expressed as percentages of positive samples in each host (the numbers of samples used for the analysis are shown in parenthesis) and different colors indicate percentages of samples positive forT. murisandB. wadsworthiaat different relative abundance ranges. Hosts with less than 20 amplicon samples are not shown.T. muris-andB. wadsworthia-related sequences co-occur in only 28 mouse gut samples as shown by the Venn diagram. For comparison, the abundance ofB. wadsworthia-positive mouse gut samples is also shown after removal of data from mice that were ‘humanized’ by receiving human feces transplants or human strain consortia.bVisualization ofTaurinivoransin a colon tissue section of a mouse (n= 1) fed a polysaccharide- and fiber-deficient diet108by FISH. TAU1151-Cy3-labeledTaurinivoranscells appear in pink and the remaining bacterial cells and tissue in blue due to DAPI-staining. The dashed line indicates the border between epithelial cells and the gut lumen. Source data are provided as a Source Data file. T. muris and B. wadsworthia use similar electron acceptors and donors, yet differ in the metabolic pathways to use them. Differential relative mRNA and protein abundances of T. muris LT0009 grown on taurine and sulfolactate suggest a differential regulation of the two organosulfonate metabolisms. 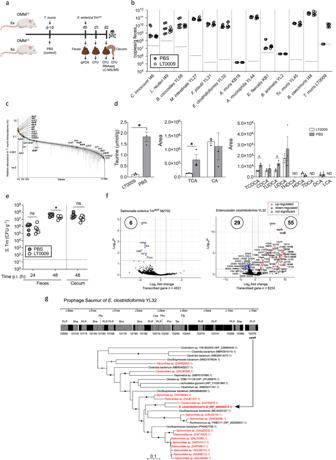Fig. 4:Taurinivorans murismainly respires taurine released from taurine-conjugated bile acids by other bacteria and slightly enhances colonization resistance againstSalmonella entericain a gnotobiotic mouse model. aSchematic outline of the gnotobiotic mouse experiment. Created with Biorender.com. Mice stably colonized with the 12-strain Oligo-Mouse-Microbiota (OMM12) were inoculated withT. murisLT0009 (n= 6 mice) or sterile phosphate-buffered saline (PBS) as control (n= 6 mice) and, after 10 days, orally and rectally infected withS. entericaTmavirM2702. Mice were sacrificed two days post infection (p.i.). Fecal samples were used for strain-specific 16 S rRNA gene-targeted quantitative PCR (qPCR). Fecal and cecal samples at 24 h and 48 h p.i. were used to analyze colony forming units (CFU) ofS. entericaTm. Fecal samples at 48 h p.i. were used for metatranscriptomics (RNAseq) and taurine and bile acids quantification (LC-MS/MS).bAbsolute abundances (16 S rRNA gene copy numbers per gram feces) of each OMM12strain and strain LT0009 on day 10 in feces of mice with and without LT0009 (PBS). Small horizontal lines indicate median values. Gray horizontal lines indicate the detection limit of each strain-specific qPCR assay.cRanked relative transcript abundance of LT0009 genes in OMM12mice fecal metatranscriptomes. Each point is the mean relative abundance of a gene and error bars correspond to the 95% confidence interval of the mean (n= 3 mice). The total number of transcribed LT0009 genes is shown (n= 1884). Genes for taurine (tpa,xsc,ald), sulfite (dsrAB, dsrC), sulfolactate (suyAB,sclC,comC) thiosulfate (sbdP, dsrE), pyruvate (por), lactate (lutABC), and hydrogen (hybA,hybC) metabolism are shown in different colors. Sulfur metabolism genes are further highlighted in bold font. Vertical dashed lines delineate the top 1%, 5%, and 10% expression rank of all 2059 protein-coding genes in the LT0009 genome.dAbsolute concentration of taurine in feces of OMM12mice treated with LT0009 (n= 3 mice) or PBS (n= 3 mice). Semi-quantitative analyses of high abundant (TCA and CA) and low abundant bile acids. Colonization of LT0009 significantly reduced the concentrations of taurine (p= 0.01), TCA (p= 0.04), TCDCA (p= 0.005), and TUDCA (p= 0.02) in the feces of OMM12mice. THDCA, TDCA, and LCA were not detected. Mean values ± SD are plotted. *p< 0.05, Student’sttest, two-sided. CA, cholic acid; CDCA, chenodeoxycholic acid; UDCA, ursodeoxycholic acid; HDCA, hyodeoxycholic acid; DCA, deoxycholic acid; LCA, lithocholic acid; prefix T indicates taurine-conjugated bile acid species; ND, not detected. e. CFU ofS. entericaTm at 24 h and 48 h p.i. in the feces and at 48 h p.i. in the cecal content. Small horizontal lines indicate median values. The dotted horizontal line shows the CFU detection limit. The asterisk indicates significant differences (p= 0.01; studentttest, two-sided) between S. enterica Tmavir CFU in mice with LT0009 and the PBS-control mice at 48 h. ns, not significant. f. Volcano plots of differential gene transcription (5% false discovery rate, DESeq2 Wald test) ofS. entericaTmavirM2702 and E. clostridioformis YL32 in OMM12mice with (n= 3 mice) and without LT0009 (n= 3 mice). Thexaxis shows log-fold-change in transcription and theyaxis shows the negative logarithm10-transformed adjustedpvalues. Blue dots show significantly downregulated genes (adjustedpvalue < 0.05, log2 fold change < −1) in mice with LT0009 and are labeled with locus tag numbers. UpregulatedE. clostridioformisYL32 prophage genes in I5Q83_10075-10390 are highlighted in bold. g. Structure of the activated prophage gene cluster ofE. clostridioformisYL32 and phylogeny of its encoded phosphoadenosine-phosphosulfate reductase (CysH). Virus- and bacteria-encoded sequences are shown in red and black, respectively. The maximum likelihood CysH tree is midpoint rooted. Ultrafast bootstrap support values equal to or >95% and 80% for the maximum likelihood tree are indicated with black and gray circles, respectively. The identity of the 61 genes in the prophage region (I5Q83_10075-10390) ofE. clostridioformisYL32 as predicted by PHASTER99. Genes encoding hypothetical proteins are in black and annotated genes are in gray. Numbers indicate the locus tag. PLP phage-like protein, Sha tail shaft, Pla plate protein, Coa coat protein, Pro protease, Por portal protein, Ter terminase, Fib fiber protein. Source data are provided as a Source Data file. However, strain LT0009 maintained a high cellular prevalence of its taurine metabolism enzymes Tpa, Ald, and Xsc independent of the used electron acceptor. Given that taurine is a largely host-derived and thus permanently available substrate in the animal gut, a predominantly constitutive expression and/or high stability of taurine-degrading proteins could sustain the fitness of T. muris in the gut ecosystem [61] . Distinct distribution patterns of Taurinivorans muris and Bilophila wadsworthia suggest different host preferences B. wadsworthia was repeatedly reported as a taurine-degrading member of the murine intestine based on molecular surveys [24] , [26] , [62] . We performed a meta-analysis to compare the presence and relative abundance of B. wadsworthia- related and T. muris -related sequences across thousands of 16 S rRNA gene amplicon datasets from the intestinal tract of diverse hosts. T. muris -related 16 S rRNA gene sequences were most often detected in the mouse gut, i.e., in 14.4% of all mouse amplicon datasets, but also present in the datasets from multiple other hosts (shrimp, pig, rat, chicken, fish, cow, humans, termites, and other insects) (Fig. 3a , Supplementary Data 4 ). In comparison, B. wadsworthia- related sequences are most widespread in the human gut, i.e., in 30.7% of human gut amplicon datasets, but are also prevalent in pig (15.8%), chicken (13.7%), and rat (9.8%) and occasionally detected in other hosts (Fig. 3a ). We also identified B. wadsworthia- related sequences in 7.5% of mouse datasets. T. muris - and B. wadsworthia- related sequences co-occurred only in 28 mouse datasets, which could be due to differential adaptation to the murine and human gut of the two organisms and/or their competitive exclusion by competition for taurine. Furthermore, we found that 82% of the B. wadsworthia -positive samples are from mice that were ‘humanized’ by receiving human feces transplants or human strain consortia [63] , [64] , [65] , [66] , which suggests a much lower prevalence of B. wadsworthia strains that are indigenous in mice. T. muris -related sequences represented >5% of the total community in 2.8% of mouse gut datasets (Fig. 3a ). Such very high relative 16 S rRNA gene abundances were more often observed in mice on high-fat diets [67] , [68] , but sporadically also in mice on standard chow and other diets (Fig. 3b ) [69] . Fig. 3: Taurinivorans muris and Bilophila wadsworthia have distinct host distribution patterns. a Occurrence and prevalence of Taurinivorans muris - and Bilophila wadsworthia -related sequences in 16 S rRNA gene amplicon datasets of human and animal guts. T. muris - and B. wadsworthia -like sequences at 97% similarity cutoff are expressed as percentages of positive samples in each host (the numbers of samples used for the analysis are shown in parenthesis) and different colors indicate percentages of samples positive for T. muris and B. wadsworthia at different relative abundance ranges. Hosts with less than 20 amplicon samples are not shown. T. muris- and B. wadsworthia- related sequences co-occur in only 28 mouse gut samples as shown by the Venn diagram. For comparison, the abundance of B. wadsworthia -positive mouse gut samples is also shown after removal of data from mice that were ‘humanized’ by receiving human feces transplants or human strain consortia. b Visualization of Taurinivorans in a colon tissue section of a mouse ( n = 1) fed a polysaccharide- and fiber-deficient diet [108] by FISH. TAU1151-Cy3-labeled Taurinivorans cells appear in pink and the remaining bacterial cells and tissue in blue due to DAPI-staining. The dashed line indicates the border between epithelial cells and the gut lumen. Source data are provided as a Source Data file. Full size image Overall, T. muris is considerably more abundant and prevalent in the mouse gut microbiome than B. wadsworthia . Notably, a mouse native B. wadsworthia strain has not yet been isolated. Our phylogenomic analysis of all de-replicated, high-quality Desulfovibrionaceae MAGs from the integrated mouse gut metagenome catalog (iMGMC) [70] revealed two MAGs form a well-supported monophyletic group with B. wadsworthia strains (Fig. 1b ). Mouse MAG iMGMC-189 has a minimum ANI of 82% and AAI of 79% to B. wadsworthia , which suggests that it represents the population genome of a new, murine Bilophila species. Mouse MAG extra-SRR7761328.52 is more distantly related and has a minimum ANI of 78% and AAI of 65% to B. wadsworthia . Both mouse MAGs encode the taurine degradation pathway ( tpa-sarD-islAB ) of B. wadsworthia (Supplementary Fig. 1 ), while the pathway for sulfolactate degradation ( slcC-comC-suyAB ) is absent in MAG extra-SRR7761328.52. In general, genes for utilization of diverse organosulfonates are widely and patchily distributed in the Desulfovibrio-Bilophila-Mailhella-Taurinivorans clade (Supplementary Fig. 1 ) [71] . Other mouse Desulfovibrionaceae that encode the capability for taurine respiration include (i) the Desulfovibrio -affiliated MAGs extra-SRR7533634.94 and iMGMC-585 with the tpa-xsc pathway and (ii) the Mailhella -related MAG extra-SRR7691169.24 with the tpa-sarD-islAB pathway (Supplementary Fig. 1 ). Taurine degradation is the main in vivo realized nutritional niche of Taurinivorans muris We next performed metatranscriptome analysis and re-analyzed published metatranscriptome datasets of gut samples from different mouse models to reveal the metabolic pathways that are most expressed by T. muris in its murine host. In our gnotobiotic model, strain LT0009 or a mock control was added to germ-free mice stably colonized with the synthetic OMM 12 community, which does not encode dsrAB-dsrC for sulfite respiration (Fig. 4a ). Strain-specific qPCR assays showed that ten OMM 12 strains and strain LT0009 colonized the mice (Fig. 4b ). Consistent with previous studies, strains A. muris KB18 and B. longum subsp. animalis YL2 were not detected [72] , [73] . Colonization of LT0009 did not affect the abundance of other strains, which indicated that LT0009 occupied a free niche in the intestinal tract of this gnotobiotic mouse model. The taurine metabolism ( tpa , ald , xsc ) and sulfite reduction ( dsrAB, dsrC ) genes were in the top 5% expression rank of all LT0009 genes (Fig. 4c ). In contrast, transcription of the putative thiosulfate transferase gene ( sbdP ) ranked at 17% and of sulfolactate degradation genes ( suyAB , slcC , comC ) ranked from 62% to 88% of all LT0009 genes (Fig. 4c ). LT0009-colonized mice showed a significant, 15-fold reduction in fecal taurine concentrations (Fig. 4d ). T. muris LT0009 thus largely occupied the vacant taurine-nutrient niche in the intestinal tract of OMM [12] mice. Metatranscriptome analyses of intestinal samples from conventional laboratory mice on various diets (e.g., high-glucose; high-fat/low-carbohydrate; low-fat/high-carbohydrate) and with different genetic backgrounds (wild-type; plin2) also showed that taurine degradation and sulfite respiration were within the top 5% of expressed LT0009 genes (Supplementary Fig. 6 ). Fig. 4: Taurinivorans muris mainly respires taurine released from taurine-conjugated bile acids by other bacteria and slightly enhances colonization resistance against Salmonella enterica in a gnotobiotic mouse model. a Schematic outline of the gnotobiotic mouse experiment. Created with Biorender.com. Mice stably colonized with the 12-strain Oligo-Mouse-Microbiota (OMM 12 ) were inoculated with T. muris LT0009 ( n = 6 mice) or sterile phosphate-buffered saline (PBS) as control ( n = 6 mice) and, after 10 days, orally and rectally infected with S. enterica Tm avir M2702. Mice were sacrificed two days post infection (p.i.). Fecal samples were used for strain-specific 16 S rRNA gene-targeted quantitative PCR (qPCR). Fecal and cecal samples at 24 h and 48 h p.i. were used to analyze colony forming units (CFU) of S. enterica Tm. Fecal samples at 48 h p.i. were used for metatranscriptomics (RNAseq) and taurine and bile acids quantification (LC-MS/MS). b Absolute abundances (16 S rRNA gene copy numbers per gram feces) of each OMM 12 strain and strain LT0009 on day 10 in feces of mice with and without LT0009 (PBS). Small horizontal lines indicate median values. Gray horizontal lines indicate the detection limit of each strain-specific qPCR assay. c Ranked relative transcript abundance of LT0009 genes in OMM 12 mice fecal metatranscriptomes. Each point is the mean relative abundance of a gene and error bars correspond to the 95% confidence interval of the mean ( n = 3 mice). The total number of transcribed LT0009 genes is shown ( n = 1884). Genes for taurine ( tpa , xs c, ald ), sulfite ( dsrAB, dsrC ), sulfolactate ( suyAB , sclC , comC ) thiosulfate ( sbdP, dsrE ), pyruvate ( por ), lactate ( lutABC ), and hydrogen ( hybA , hybC ) metabolism are shown in different colors. Sulfur metabolism genes are further highlighted in bold font. Vertical dashed lines delineate the top 1%, 5%, and 10% expression rank of all 2059 protein-coding genes in the LT0009 genome. d Absolute concentration of taurine in feces of OMM 12 mice treated with LT0009 ( n = 3 mice) or PBS ( n = 3 mice). Semi-quantitative analyses of high abundant (TCA and CA) and low abundant bile acids. Colonization of LT0009 significantly reduced the concentrations of taurine ( p = 0.01), TCA ( p = 0.04), TCDCA ( p = 0.005), and TUDCA ( p = 0.02) in the feces of OMM 12 mice. THDCA, TDCA, and LCA were not detected. Mean values ± SD are plotted. * p < 0.05, Student’s t test, two-sided. CA, cholic acid; CDCA, chenodeoxycholic acid; UDCA, ursodeoxycholic acid; HDCA, hyodeoxycholic acid; DCA, deoxycholic acid; LCA, lithocholic acid; prefix T indicates taurine-conjugated bile acid species; ND, not detected. e. CFU of S. enterica Tm at 24 h and 48 h p.i. in the feces and at 48 h p.i. in the cecal content. Small horizontal lines indicate median values. The dotted horizontal line shows the CFU detection limit. The asterisk indicates significant differences ( p = 0.01; student t test, two-sided) between S. enterica Tmavir CFU in mice with LT0009 and the PBS-control mice at 48 h. ns, not significant. f. Volcano plots of differential gene transcription (5% false discovery rate, DESeq2 Wald test) of S. enterica Tm avir M2702 and E. clostridioformis YL32 in OMM 12 mice with ( n = 3 mice) and without LT0009 ( n = 3 mice). The x axis shows log-fold-change in transcription and the y axis shows the negative logarithm10-transformed adjusted p values. Blue dots show significantly downregulated genes (adjusted p value < 0.05, log2 fold change < −1) in mice with LT0009 and are labeled with locus tag numbers. Upregulated E. clostridioformis YL32 prophage genes in I5Q83_10075-10390 are highlighted in bold. g. Structure of the activated prophage gene cluster of E. clostridioformis YL32 and phylogeny of its encoded phosphoadenosine-phosphosulfate reductase (CysH). Virus- and bacteria-encoded sequences are shown in red and black, respectively. The maximum likelihood CysH tree is midpoint rooted. Ultrafast bootstrap support values equal to or >95% and 80% for the maximum likelihood tree are indicated with black and gray circles, respectively. The identity of the 61 genes in the prophage region (I5Q83_10075-10390) of E. clostridioformis YL32 as predicted by PHASTER [99] . Genes encoding hypothetical proteins are in black and annotated genes are in gray. Numbers indicate the locus tag. PLP phage-like protein, Sha tail shaft, Pla plate protein, Coa coat protein, Pro protease, Por portal protein, Ter terminase, Fib fiber protein. Source data are provided as a Source Data file. Full size image Free taurine in the murine intestine largely derives from microbial deconjugation of host-derived taurine-conjugated bile acids [74] , [75] . LT0009 does not encode bile salt hydrolase (BSH) genes and thus likely depends on other gut microbiota members to liberate taurine from taurine-conjugated bile acids. BSH genes are encoded across diverse bacterial taxa in the human and mouse gut [74] , [76] , [77] . In agreement with previous studies of bile acid transformations in the OMM 12 model [78] , [79] , we identified BSH genes in seven OMM 12 strains (Supplementary Data 5 ). BSH gene transcription increased in Enterocloster clostridioformis YL32, Enterococcus faecalis KB1, Bacteroides caecimuris I48, and Muribaculum intestinale YL27, and decreased in Limosilactobacillus reuteri I49, but not significantly (Supplementary Data 5 and 6 ). Bile acid deconjugation by some of these OMM 12 strains has been confirmed in vitro [79] . Specifically, E. faecalis KB1, B. caecimuris I48, M. intestinale YL27, and Bifidobacterium animalis YL2 tested positive for deconjugation of taurine-conjugated deoxycholic acid, while E. clostridioformis YL32 either tested negative or was inhibited by addition of bile acids. The down-regulation of the BSH gene in L. reuteri I49 is consistent with the in vitro deconjugation capacity of this strain for glycine-conjugated deoxycholic acid but not for taurine-conjugated deoxycholic acid [79] and the generally lower abundance of glycine-conjugated bile acids in rodents [75] . We thus hypothesized that taurine degradation by LT0009 could provide a positive feedback mechanism on the expression of BSHs for taurine-conjugated bile acid deconjugation in the OMM 12 model. In support of this hypothesis, the abundance of several taurine-conjugated bile acids was significantly reduced in feces of OMM 12 mice with LT0009 (Fig. 4d ). Additional in vitro growth experiments and mono- and co-colonization experiments with germ-free mice confirmed that T. muris LT0009 can not grow on taurine-conjugated bile acids in pure culture and is strictly dependent on bile acid-deconjugating bacteria for successful colonization of the mouse gut (Supplementary Information, Supplementary Figs. 7 and 8 ). Thiosulfate is presumably a constantly present electron acceptor for microbial respiration in the mammalian gut as it is generated by mitochondrial H 2 S oxidation in the gut epithelium [1] . Mitochondrial sulfide oxidation mainly takes place apically in the crypts of human colonic tissue at the interface to the gut microbiota [80] . The amount of thiosulfate supplied into the gut lumen depends on epithelial H 2 S metabolism [1] , [80] . The expression level of the putative SbdP thiosulfate transferase of T. muris ranked relatively high with 15–24% of all LT0009 genes across all gut samples from the various mouse models (Fig. 4c , Supplementary Fig. 6 ). However, the function of this protein remains unconfirmed as its expression was not differentially upregulated in the thiosulfate-metabolizing T. muris pure culture (Fig. 2a, d , Supplementary Data 1 ). In vivo, taurine respiration, and potentially thiosulfate respiration, are likely fueled by pyruvate, H 2 , and lactate as electron donors, as expression of genes for their oxidation ranked at 5–7% ( por ), 1.5–9.1% ( hybAC ), and 2.5–31% ( lutABC , lutP ) of all LT0009 genes across all mouse gut metatranscriptomes, respectively (Fig. 4c , Supplementary Fig. 6 ). Together with the highly specialized fundamental physiology of the T. muris pure culture (Fig. 2 ), these results strongly suggest that taurine is the predominant electron acceptor for energy conservation of T. muris in the murine intestinal tract. Taurinivorans muris LT0009 slightly increased colonization resistance against S. enterica and increased transcriptional activity of a sulfur metabolism gene-encoding prophage in a gnotobiotic mouse model The human enteropathogen S. enterica Tm can invade and colonize the intestinal tract by utilizing various substrates for respiratory growth that are available at different infection stages [81] . The gnotobiotic OMM 12 mouse model provides intermediate colonization resistance against S. enterica Tm [72] and is widely used as a model system of modifiable strain composition for investigating the causal involvement of cultivated mouse microbiota members in diverse host diseases and phenotypes [82] . Yet, a bacterial isolate from the mouse gut with proven dissimilatory sulfidogenic capacity was unavailable until now [83] . T. muris has fundamental physiological features that could, on the one hand, contribute to colonization resistance against S. enterica Tm by direct competition for pyruvate [84] , lactate [85] , H 2 [86] , formate [87] , and host-derived thiosulfate [87] , [88] . On the other hand, T. muris could also promote S. enterica Tm expansion during inflammation by fueling tetrathionate production through enhanced intestinal sulfur metabolism [18] , [89] . Here, we investigated the impact of T. muris LT0009 during the initial niche invasion of S. enterica Tm using an avirulent, non-colitogenic strain [90] . Compared to OMM 12 mice without LT0009, mice colonized with the OMM 12 and LT0009 had a slightly reduced load of S. enterica Tm at 48 p.i. that was significant in feces but not in cecum (Fig. 4e ). Comparative metatranscriptome analysis did not provide evidence for H 2 S-mediated inhibition of S. enterica Tm respiration, as shown for other enteropathogens [91] , or any other mechanism of direct interaction. Six S. enterica Tm genes were differentially expressed, i.e., significantly downregulated, in the presence of strain LT0009 (Fig. 4f , Supplementary Data 6 ). Three of the six genes are involved in transport and metabolism of galactonate ( d -galactonate transporter DgoT, D-galactonate dehydratase DgoD, 2-dehydro-3-deoxy-6-phosphogalactonate aldolase DgoA), which is produced by some bacteria as an intermediate in D-galactose metabolism and is also present in mammalian tissue and body secretions [92] . D-galactonate catabolism capability was suggested as a distinguishing genetic feature of intestinal Salmonella strains compared to extraintestinal serovars, with serovars Typhi, Paratyphi A, Agona, and Infantis lacking genes for utilizing D-galactonate as a sole carbon source [93] . The putative D-galactonate transporter DgoT in Salmonella enterica serovar Choleraesuis was identified as a virulence determinant in pigs [94] . The OMM 12 strains and LT0009 do not encode the DgoTDAKR galactonate pathway. The significance of galactonate for S. enterica Tm gut colonization and competition remains to be elucidated. Colonization of T. muris LT0009 in the gnotobiotic mice had variable impact on the differential gene expression pattern of the OMM 12 members (Fig. 4f , Supplementary Fig. 9 , Supplementary Data 6 ). While gene expression was not significantly affected in L. reuteri I49, E. clostridioformis YL32 was most affected with 84 differentially expressed genes (55 upregulated and 29 downregulated) (Fig. 4f ). 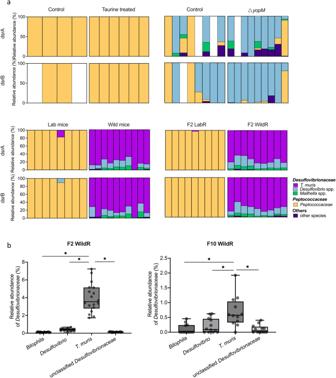Fig. 5:Taurinivorans murisis the dominant sulfidogen in wild-mouse-microbiota-derived wildR mice that provided H2S-mediated protection againstKlebsiella pneumoniae. Re-analysis of mouse gut metagenome and 16 S rRNA gene amplicon data from Stacy et al.37.aIdentity and relative abundance ofdsrAB-encoding taxa in different mouse models. Relative abundance was calculated with mappeddsrAanddsrBread counts. Samples with less than ten total mapped read counts were not displayed. Each column shows a sample from an individual mouse. Taurine-treated mice: specific-pathogen-free (SPF) mice that received taurine in drinking water and showed enhanced resistance toKlebsiella pneumoniaeandCitrobacter rodentium; ΔyopMmice: SPF mice that were previously infected with the attenuated strain ΔyopMof the food-borne pathogenYersinia pseudotuberculosisand showed enhanced resistance toK. pneumoniae; SPF mice were used as control for taurine-treated and ΔyopMmice; lab mice: laboratory SPF mice; wild mice: wild-caught mice; F2 LabR mice: the second generation offspring of SPF mice whose germ-free founders received the microbiota of labR mice; F2 wildR mice: the second generation offspring of SPF mice whose germ-free founders received the microbiota of wild mice and showed enhanced resistance toK. pneumoniae.bRelative 16 S rRNA gene abundance ofDesulfovibrionaceaespecies in the 2nd (animal. Ordinary one-way ANOVA with Holm-Sidak’s multiple comparisons test, *p< 0.05. Source data are provided as a Source Data file. 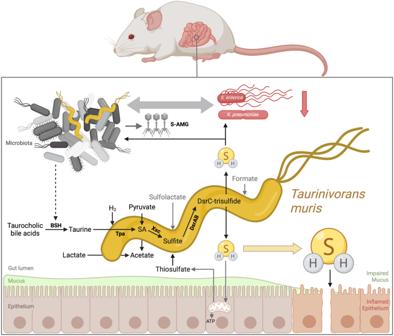Fig. 6: Sulfur energy metabolism and proposed interaction scheme ofTaurinivorans murisin the mouse gut. T. murismainly utilizes taurine as the main electron acceptor for anaerobic respiration in the gut but is also capable of thiosulfate and sulfolactate respiration. Pyruvate, lactate, and likely hydrogen are the main electron donors ofT. muris, while formate could also be used. Taurine is cleaved from host-derived taurine-conjugated bile acids by other gut bacteria via bile salt hydrolase (BSH). Thiosulfate derives from mitochondrial oxidation of H2S in the gut epithelium.T. murisproduces H2S from taurine via pyruvate-dependent taurine transaminase (Tpa), sulfoacetaldehyde (SA) acetyltransferase (Xsc), and dissimilatory sulfite reductase (DsrAB). H2S can have various effects on the gut microbiota and host health. For example, excess H2S can impair mucus integrity3. H2S can enhance resistance against enteropathogens by directly inhibiting enzymes in aerobically respiringKlebsiella pneumoniae37.T. muriscould further impact microbial interactions and intestinal metabolism by stimulating the transcriptional activity of prophages that encode auxiliary metabolic genes, such as those involved in sulfur metabolism (S-AMG)100. Created with Biorender.com. Most of the significantly upregulated genes ( n = 41) in E. clostridioformis YL32 are clustered in a large genomic region (I5Q83_10075-10390) that encoded various phage gene homologs and was identified as a prophage using PHASTER (Fig. 4g ). This prophage, named YL32-pp-2.059, Saumur, is among a set of thirteen previously identified prophages of the OMM 12 consortium that represent novel viruses, were induced under various in vitro and/or in vivo conditions, and constitute the temporally stable viral community of OMM 12 mice [95] . We show that colonization of LT0009 in the OMM 12 mouse model selectively enhanced the transcriptional activity of the E. clostridioformis YL32 prophage Saumur, which carries a gene (I5Q83_10375) for phosphoadenosine-phosphosulfate reductase (CysH) that functions in the assimilatory sulfate reduction pathway of many bacteria (Fig. 4g ). Various organosulfur auxiliary metabolic genes, particularly cysH , are widespread in environmental and human-associated viromes, which suggests viruses augment sulfur metabolic processes in these environments, including the gut [96] . Addition of sulfide to a Lactococcus lactis strain culture was shown to increase production of viable particles of its phage P087 [96] , but it is unknown if H 2 S can activate prophages. We speculated that T. muris LT0009 could impact intestinal sulfur homeostasis not only via its own sulfur metabolism but also by activation of the sulfur metabolism gene-expressing phage Saumur in E. clostridioformis YL32, possibly via H 2 S. Growth tests with the pure culture of E. clostridioformis YL32 at two physiologically relevant sulfide concentrations demonstrated reduced growth at a high sulfide concentration (Supplementary Information, Supplementary Fig. 10 ). However, quantification of host and prophage genes did not show activation of the prophage Saumur under the tested condition. How prophage Saumur is activated and if its in vivo activity contributes to protection from S. enterica Tm thus remains subject of further study. Taurinivorans muris is the dominant sulfidogen in a wild-mouse-microbiota mouse model that provided H 2 S-mediated protection against Klebsiella pneumoniae Expansion of sulfidogenic bacteria and the tpa-xsc-dsr pathway in the metagenome fueled by host-derived taurine was previously shown to contribute to protection against the enteropathogen Klebsiella pneumoniae and Citrobacter rodentium in different mouse models; with sulfide-mediated inhibition of aerobic respiration by pathogens being proposed as a generic protective mechanism [91] . Here, we have re-analyzed the 16 S rRNA gene amplicon data and the reads of dsrAB , the sulfite reductase marker genes for sulfide production [97] , from the metagenome data of this study. We identified T. muris as the dominant deltaproteobacterium ( Desulfobacterota ) and dsrAB -containing member of the microbiota of wild mice and the wild-mouse-microbiota (wildR) mouse model, but not in the other mouse models (Fig. 5 ). Given that taurine respiration via the sulfidogenic tpa-xsc-dsr pathway is the main energy niche of T. muris in the mouse gut (Fig. 4c , Supplementary Fig. 6 ), the enhanced resistance against Klebsiella pneumoniae in the wildR mouse model [91] was thus primarily due to the activity of T. muris . Sulfide-mediated protection against Klebsiella pneumoniae and Citrobacter rodentium in the other mouse models, i.e., taurine-supplemented and Δ yopM mice, was not provided by T. muris but by other sulfidogens (Fig. 5 ) [91] . Fig. 5: Taurinivorans muris is the dominant sulfidogen in wild-mouse-microbiota-derived wildR mice that provided H 2 S-mediated protection against Klebsiella pneumoniae . Re-analysis of mouse gut metagenome and 16 S rRNA gene amplicon data from Stacy et al. [37] . a Identity and relative abundance of dsrAB -encoding taxa in different mouse models. Relative abundance was calculated with mapped dsrA and dsrB read counts. Samples with less than ten total mapped read counts were not displayed. Each column shows a sample from an individual mouse. Taurine-treated mice: specific-pathogen-free (SPF) mice that received taurine in drinking water and showed enhanced resistance to Klebsiella pneumoniae and Citrobacter rodentium ; Δ yopM mice: SPF mice that were previously infected with the attenuated strain Δ yopM of the food-borne pathogen Yersinia pseudotuberculosis and showed enhanced resistance to K. pneumoniae ; SPF mice were used as control for taurine-treated and Δ yopM mice; lab mice: laboratory SPF mice; wild mice: wild-caught mice; F2 LabR mice: the second generation offspring of SPF mice whose germ-free founders received the microbiota of labR mice; F2 wildR mice: the second generation offspring of SPF mice whose germ-free founders received the microbiota of wild mice and showed enhanced resistance to K. pneumoniae . b Relative 16 S rRNA gene abundance of Desulfovibrionaceae species in the 2nd (animal. Ordinary one-way ANOVA with Holm-Sidak’s multiple comparisons test, * p < 0.05. Source data are provided as a Source Data file. Full size image Taurinivorans muris LT0009 provides a core function in gnotobiotic mouse models Dissimilatory sulfur metabolism with the production of H 2 S is a core metabolic capability of the mammalian gut microbiota that is carried out by specialized bacteria [71] , [98] . As in humans and other animals, bacteria of the phylum Desulfobacterota (formerly Deltaproteobacteria ), specifically of the Desulfovibrio-Mailhella-Bilophila lineage [35] , are important sulfidogens in the mouse gut and appear to be more abundant in wild mice compared to untreated laboratory mice [99] , [100] . However, the diversity of sulfidogenic microorganisms and their metabolic pathways in the intestinal tract of non-human animals, including mice that represent important experimental models, remain insufficiently understood. A mouse gut-derived Desulfobacterota strain ( Desulfovibrio strain MGBC000161) was recently isolated, but not physiologically characterized [99] . Here, we contribute the sulfidogenic strain LT0009, representing the newly proposed genus Taurinivorans , to the growing collection of publicly available bacterial strains from the mouse [83] , [99] . We further describe the fundamental metabolic properties and realized lifestyle of Taurinivorans muris , which relies on taurine as the primary electron acceptor for energy conservation in vivo and can contribute to the protective effect of the commensal mouse gut microbiota against S. enterica and K. pneumoniae (Fig. 6 ). In addition to direct inhibition of aerobic respiration of pathogens by H 2 S as shown previously [91] , indirect, not yet fully resolved resistance mechanisms, which are dependent on the respective pathogen and composition of the resident microbiota, can be at play. Presence of T. muris selectively increased transcription of a phosphoadenosine-phosphosulfate reductase (CysH)-encoding prophage in another bacterium and could thereby modulate microbiome functions. T. muris strain LT0009 is currently the only murine Desulfobacterota isolate with a physiologically proven dissimilatory sulfur metabolism and thus significantly extends the experimental options to study the role of sulfidogenic bacteria in gnotobiotic mouse models. Fig. 6: Sulfur energy metabolism and proposed interaction scheme of Taurinivorans muris in the mouse gut. T. muris mainly utilizes taurine as the main electron acceptor for anaerobic respiration in the gut but is also capable of thiosulfate and sulfolactate respiration. Pyruvate, lactate, and likely hydrogen are the main electron donors of T. muris , while formate could also be used. Taurine is cleaved from host-derived taurine-conjugated bile acids by other gut bacteria via bile salt hydrolase (BSH). Thiosulfate derives from mitochondrial oxidation of H 2 S in the gut epithelium. T. muris produces H 2 S from taurine via pyruvate-dependent taurine transaminase (Tpa), sulfoacetaldehyde (SA) acetyltransferase (Xsc), and dissimilatory sulfite reductase (DsrAB). H 2 S can have various effects on the gut microbiota and host health. For example, excess H 2 S can impair mucus integrity [3] . H 2 S can enhance resistance against enteropathogens by directly inhibiting enzymes in aerobically respiring Klebsiella pneumoniae [37] . T. muris could further impact microbial interactions and intestinal metabolism by stimulating the transcriptional activity of prophages that encode auxiliary metabolic genes, such as those involved in sulfur metabolism (S-AMG) [100] . Created with Biorender.com. Full size image Supplementary Information provides further details on the methods described below. All animal experiments complied with ethical regulations and were approved by local authorities in Germany (Regierung von Oberbayern; ROB-55.2-2532.Vet_02-20-84) or by national Austrian authorities (Bundesministerium für Bildung, Wissenschaft und Forschung; BMWF-66.006/0032-WF/V/3b/2014). Isolation of strain LT0009 and growth experiments Intestinal contents of wild-type C57BL/6 mice were used as inocula for the enrichment cultures. A modified Desulfovibrio medium was used to isolate strain LT0009 with taurine as electron acceptor and lactate and pyruvate as electron donors and for further growth experiments. Consumption of taurine and lactate and production of H 2 S and SCFA were measured [71] . Strain LT0009 was tested for optimal taurine concentration and growth with/without pyruvate supplementation, different electron donors and acceptors, optimal pH and temperature, and growth on taurocholic acid. Microscopy Gram staining of the LT0009 isolate was performed using a Gram staining kit according to the manufacturer’s instruction (Sigma Aldrich, 77730-1KT-F), and its cellular morphology was imaged with a scanning electron microscope (JSM-IT300, JOEL). A probe was designed, tested, and applied for fluorescence in situ hybridization (FISH)-based microscopy of the genus Taurinivorans (Supplementary Data 2 , Supplementary Fig. 2 ). Genome sequencing and comparative sequence analyses The complete genome of strain LT0009 was determined by combined short- (Illumina) and long-read (Nanopore) sequencing. The automated annotation of the genome was manually curated for genes of interest, focusing on energy metabolism. Phylogenomic analyses comprised treeing with 43 concatenated marker sequences [34] and calculating average amino acid identities (AAI) and whole-genome average nucleotide identities (gANI). Additional phylogenetic trees were calculated with LT0009 using sequences of the 16 S rRNA gene and selected sulfur metabolism proteins or genes. Source information of 16 S rRNA gene reference sequences was manually compiled from the National Center for Biotechnology Information (NCBI) Sequence Read Archive (SRA) entries (Supplementary Data 7 ). Differential proteomics and transcriptomics The total proteomes and transcriptomes of strain LT0009 grown with taurine, sulfolactate, or thiosulfate as electron acceptor and lactate/pyruvate as electron donor were determined and compared. Analyses of publicly available 16 S rRNA sequence data The occurrence and prevalence of Taurinivorans muris - and Bilophila wadsworthia -related 16 S rRNA gene sequences were analyzed across 123,723 amplicon datasets from gut samples, including 81,501 with host information. Further information on mouse studies with at least 20 samples that were positive for B. wadsworthia was manually compiled from the NCBI SRA entries or the corresponding publications (Supplementary Data 8 ). LT0009-centric gut metatranscriptome analyses of laboratory mice Cecal and fecal metatranscriptomes from a high-glucose diet experiment in mice (HG study) (JMF project JMF-2101-5) were analyzed for LT0009 gene expression. Mouse experiments were conducted following protocols approved by Austrian law (BMWF-66.006/ 0032-WF/V/3b/2014). Additionally, mouse gut metatranscriptomes from a previous study were analyzed for LT0009 gene expression (Plin2 study) [101] . Sequence data ( PRJNA379425 ) derived from eight-week-old C57BL/6 wild-type and Perilipin2-null (Plin2) mice fed high-fat/low-carbohydrate or low-fat/high-carbohydrate diets. Analyses of 16 S rRNA gene amplicon and metagenome data from Stacy et al. 2021 Metagenome and selected 16 S rRNA gene amplicon sequencing data of mouse models [91] , [102] that was shown in a previous study [91] to provide enhanced H 2 S-mediated colonization resistance against the enteropathogens Klebsiella pneumoniae and/or Citrobacter rodentium were re-analyzed. Gnotobiotic oligo-mouse-microbiota mouse experiment Animal experiments were approved by the local authorities (Regierung von Oberbayern; ROB-55.2-2532.Vet_02-20-84). Mice were housed in flexible film isolators (North Kent Plastic Cages) or Han-gnotocages (ZOONLAB) under germ-free conditions. The mice were supplied with autoclaved ddH 2 O and Mouse-Breeding complete feed for mice (Ssniff) ad libitum . Twelve gnotobiotic C57BL/6 mice stably colonized with the 12-strain Oligo-Mouse-Microbiota (OMM 12 ) community [72] were used for the animal experiment. OMM 12 mice ( n = 6) were orally (50 µl) and rectally (100 µl) inoculated with strain LT0009. The control OMM 12 mouse group ( n = 6) was treated with the same volume of sterile 1x phosphate-buffered saline. After 10 days, the mice were infected with the human enteric pathogen Salmonella enterica serovar Typhimurium (avirulent S. enterica Tm strain M2702; 5×10 7 c.f.u.) and sacrificed two days post infection (p.i.). Fecal microbiota composition was determined by strain-specific qPCR assays [72] , including a newly developed assay for strain LT0009. Abundance of viable S. enterica Tm in feces and cecal content was determined by plating. Fecal samples from day two p.i. were used for (i) metatranscriptome sequencing ( n = 3 for each group) at the Joint Microbiome Facility (JFM) of the Medical University of Vienna and the University of Vienna (JMF project JMF-2104-01) and (ii) taurine and bile acids quantification ( n = 3 for each group). Mono- and co-colonization experiments in germ-free mice Animal experiments were approved by the local authorities (Regierung von Oberbayern; ROB-55.2-2532.Vet_02-20-84). Seven female germ-free C57BL/6 mice were mono-associated with strain LT0009 ( n = 4) or co-colonized with strain LT0009, Bacteroides caecimuris I48, and Enterococcus faecalis KB1 ( n = 3) by gavage. Fecal samples were collected three and seven days after inoculation for strain-specific qPCR. All mice were sacrificed 10 days after initial inoculation. Intestinal content from ileum, cecum, colon, and feces was used for strain-specific qPCR and taurine and bile acids quantification. Bile acids and taurine quantification in mouse gut content Metabolites were extracted from homogenized and dried gut content and fecal samples using methanol/acetonitrile/H 2 O (40:40:20; v:v:v) and reconstituted with (ACN/H 2 O, 50:50, v-v). Targeted LC-MS/MS analysis was performed on a Dionex Ultimate 3000 UHPLC (Thermo) system coupled to a TSQ Vantage triple quadrupole mass spectrometer (Thermo) via an electrospray ionization interface in negative polarity mode [103] . Each sample was measured in triplicate. The raw files obtained from the LC-MS/MS experiments were processed and quantified using the Skyline software [104] . The absolute concentrations of taurine and selected bile acids were calculated employing a dilution series of matrix samples spiked with reference standards of the analytes. Growth experiment of E. clostridioformis E. clostridioformis YL32 was grown anaerobically in the brain-heart-infusion medium at 37 °C. Growth was monitored by spectrophotometric measurement of the optical density at 600 nm (OD 600 ). Sodium sulfide (Na 2 S) was added to a final concentration of 0.5 mM or 5 mM. Sulfide was quantified as mentioned above. Host and prophage genes of strain YL32 were quantified by droplet digital PCR (ddPCR) (Supplementary Data 9 ). Statistics and reproducibility All growth experiments were conducted with independent biological replicates and all replications revealed similar results. No statistical method was used to predetermine the sample size. No data were excluded from the analyses. The experiments were not randomized. The investigators were not blinded to allocation during experiments and outcome assessment. Reporting summary Further information on research design is available in the Nature Portfolio Reporting Summary linked to this article.